Isotopic composition of oceanic dissolved black carbon reveals non-riverine source A portion of the charcoal and soot produced during combustion processes on land (e.g., wildfire, burning of fossil fuels) enters aquatic systems as dissolved black carbon (DBC). In terms of mass flux, rivers are the main identified source of DBC to the oceans. Since DBC is believed to be representative of the refractory carbon pool, constraining sources of marine DBC is key to understanding the long-term persistence of carbon in our global oceans. Here, we use compound-specific stable carbon isotopes (δ 13 C) to reveal that DBC in the oceans is ~6‰ enriched in 13 C compared to DBC exported by major rivers. This isotopic discrepancy indicates most riverine DBC is sequestered and/or rapidly degraded before it reaches the open ocean. Thus, we suggest that oceanic DBC does not predominantly originate from rivers and instead may be derived from another source with an isotopic signature similar to that of marine phytoplankton. Fire regimes are increasingly influenced by human activity and anthropogenic climate change [1] . The incomplete combustion of organic matter during vegetation fires and the burning of fossil fuels generates fire-derived or pyrogenic carbon, here referred to as black carbon (BC). Vegetation fires are the predominant source of terrestrial BC (~260 Tg-C yr −1 ) [2] , [3] where it is estimated that >90% of the BC produced remains on-site [3] , [4] . A relatively small portion of terrestrial BC is emitted to the atmosphere as pyrogenic aerosols (8–17 Tg-C yr −1 ) which are primarily derived from fossil fuel combustion [5] . Regardless of its formation conditions, BC is carbon-rich compared to its unburned organic precursor material [6] . Charring results in the thermal condensation of biomolecular structures, thereby altering the reactivity of the precursor organic material. Thermal alteration of biomass increases its recalcitrance, leading to longer environmental residence times which has implications when including BC in global carbon budgets [5] , [7] . BC deposited on the landscape becomes incorporated into soils to comprise ~14% of soil organic carbon stocks globally [8] . Soil BC is then mobilized to inland waters via wind, erosion, and/or leaching processes [9] , serving as a continuous source of fire-derived carbon to aquatic systems [10] . In natural waters, BC occurs in both dissolved and particulate forms [10] and factors controlling the lateral transport of soil BC to inland waters are still being refined [9] . However, current estimates suggest roughly half of total BC entering waterways occurs as dissolved BC (DBC) [11] , [12] . DBC is one of the most prevalent organic molecular classes that has been quantified in the global ocean, where it occurs at concentrations between 600 and 810 nM-C, equivalent to ~2% of total DOC [13] , [14] . In terms of mass flux, rivers are the largest identified source of DBC to the ocean [10] . The annual flux of riverine DBC to the oceans (27 Tg-C yr −1 ) [11] would replace the standing stock of oceanic DBC (14 Pg-C) [13] , [14] within ~500 years. This estimate is considerably shorter than the apparent age of DBC measured in either the surface or deep ocean (4800 and 23,000 14 C years, respectively) [14] . Thus, assuming riverine DBC is of near-modern age [14] , [15] , significant removal of riverine DBC needs to occur in order for flux- and 14 C-derived turnover times to match, even if rivers were the only source of oceanic DBC. The same discrepancy has been noted for bulk DOC, with riverine inputs capable of replacing the entire oceanic DOC pool within ~2600 years, yet radiocarbon analyses suggest the average age of oceanic DOC is 4000–6000 14 C years [16] , [17] , [18] . Although riverine DOC could replace the oceanic DOC pool approximately two times over, biomarker and stable carbon isotope data indicate that oceanic DOC contains minimal amounts of terrestrial DOC and is instead dominated by autochthonous, marine DOC [16] , [19] . Stable carbon isotopic signatures of humics isolated from oceanic DOC are also consistent with a marine source [20] , further supporting the conclusion that terrestrial DOC is efficiently removed from the ocean. Compared to previous research on bulk DOC, isotopic studies of DBC are few. Previously reported DBC δ 13 C values include only one coastal sample (~−24‰) and two river samples (~−29‰) [21] . Although these data were limited, the observed isotopic discrepancy suggested coastal DBC may have a different source than, or be a degraded (altered) version of riverine DBC and raised the question as to whether this was a local or global phenomenon. Thus, in the current study, we used compound-specific δ 13 C to probe the persistence of riverine DBC in the open ocean within a globally relevant sample set. If rivers were not the primary source of DBC in the ocean, then we would expect the δ 13 C signature of oceanic DBC to be different from that of rivers (~−29‰) [21] . If the null hypothesis was upheld, then oceanic DBC would exhibit δ 13 C signatures similar to that of riverine DBC. To test this hypothesis, water samples were collected from five major world rivers (Amazon, Congo, Northern Dvina, Kolyma, and Mississippi; total n = 12) and from the Pacific ( n = 5) and Atlantic Oceans ( n = 4) (Fig. 1 ). The sampled rivers deliver ~24% of freshwater discharge, ~17% of DOC [17] and therefore ~17% of DBC [11] to the oceans. The rivers vary in their DOC composition, land use, catchment area, geographical location, and climate, thereby capturing a wide range of potential terrestrial DBC sources and isotopic signatures [22] , [23] , [24] , [25] , [26] . Ocean samples were chosen to capture globally representative water masses and gradients in bulk DOC quality and source [16] . DOC was isolated by solid phase extraction (SPE-DOC) [27] . DBC was then measured in SPE-DOC by oxidizing condensed aromatics to individual benzenehexacarboxylic acid (B6CA) and benzenepentacarboxylic acid (B5CA) products [28] . Molecular markers B6CA and B5CA are the most dominant benzenepolycarboxylic acids (BPCAs) and are presumed to be exclusively of pyrogenic origin [29] . Individual BPCAs were then resolved, quantified, and isotopically characterized (BPCA-specific δ 13 C) to determine DBC δ 13 C values [21] . These data are presented and used to test the hypothesis that DBC found in the oceans is not isotopically consistent with DBC from rivers. Fig. 1 Map showing sites sampled for the current study. Green shaded regions denote river catchment margins. Blue stars indicates Atlantic and Pacific Ocean sampling locations. Base map was drawn using the Ocean Data View software package [72] Full size image 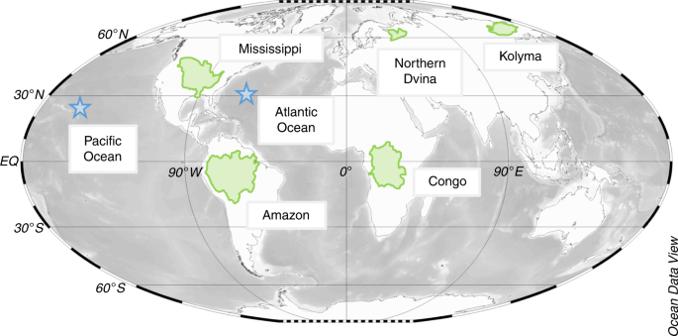Fig. 1 Map showing sites sampled for the current study. Green shaded regions denote river catchment margins. Blue stars indicates Atlantic and Pacific Ocean sampling locations. Base map was drawn using the Ocean Data View software package72 Riverine and oceanic DBC stable carbon isotopic signatures The DOC and DBC concentrations captured by our riverine sample set varied by an order of magnitude (247–1310 and 19–115 μM-C, respectively; Table 1 ), spanning the range observed for large fluvial systems globally [11] . On average, riverine B6CA and B5CA were depleted in 13 C and similar in isotopic composition to SPE-DOC (Table 1 ; Fig. 2 ), consistent with both DBC and DOC in rivers deriving from the same source [2] , [7] . Mean δ 13 C values for riverine B6CA and B5CA were −30.77 ± 1.51‰ and −29.44 ± 2.00‰, respectively. BPCA-specific δ 13 C values did not significantly vary among rivers (B6CA, p = 0.30; B5CA, p = 0.48; Table 1 ). However, SPE-DOC δ 13 C values were statistically different among some rivers ( p = 0.0004). The significant result for SPE-DOC δ 13 C values and lack thereof for BPCA-specific δ 13 C values may have been driven by the increased precision of bulk (derived from elemental analysis) versus compound-specific (derived from liquid chromatography) isotopic measurements (Table 1 ). As previously observed for bulk DOC [30] , variations in SPE-DOC δ 13 C values among rivers could also be explained, in part, by considering the types of vegetation which serve as the source of DOC in each watershed. The δ 13 C composition of plants depends on its photosynthetic pathway for fixing atmospheric carbon. Plants utilizing the globally dominant C3 pathway (e.g., woody vegetation and most vascular plants) results in biomass that is relatively depleted in 13 C (−22‰ to −30‰), whereas plants fixing carbon following the C4 pathways (e.g., corn, sugarcane, and some grasses) results in biomass that is more 13 C-enriched (−10‰ to −14‰) [31] , [32] . The rainforest-dominated Amazon River catchment exported SPE-DOC that was most depleted in 13 C, whereas the Mississippi, with increased proportions of grassland and agriculture [33] , exported SPE-DOC that was ~2‰ more enriched in 13 C (Table 1 ). The Congo River watershed is roughly half forested and half grassland [34] , yielding intermediate SPE-DOC δ 13 C values (Table 1 ). SPE-DOC exported by the Northern Dvina River in the Arctic, which primarily drains peat lowlands [35] , had statistically similar δ 13 C values as the equatorial Congo River SPE-DOC ( p = 0.09; Table 1 ). Although the reason for this was not specifically investigated, isotopic similarities between the Northern Dvina and Congo suggests SPE-DOC in each river derives from a 13 C-depleted terrestrial organic matter source. Since differences in discharge could drive variations in DBC isotopic composition, we also compared multiple samples collected across the hydrograph from the Congo and Northern Dvina Rivers. The Congo River is a low latitude, tropical river with a relatively stable hydrological regime [36] . In contrast, the high latitude Northern Dvina River exhibits strong seasonal hydrology, where discharge peaks during the spring freshet and is accompanied by high DOC concentrations [24] . Throughout the sampling period, concentrations of DOC and DBC increased by a factor of two in the Congo River and by a factor of three in the Northern Dvina River (Table 1 ). However, δ 13 C values for SPE-DOC, B6CA, and B5CA were remarkably consistent (SD < 1‰; Table 1 ). These results suggest that the isotopic composition of DBC derived from global rivers is relatively constant, remaining consistently depleted in 13 C regardless of land cover or hydrologic regime, and indicates that DBC is derived from similar source vegetation as SPE-DOC. Thus, the δ 13 C signature of BPCAs in rivers appear to be a faithful proxy for the source vegetation that presumably burnt to yield the DBC. Table 1  Concentrations, qualitative ratios, and stable carbon isotopic values (δ 13 C) of DOC, DBC, and BPCA molecular markers in rivers the ocean Full size table Fig. 2 Riverine and oceanic stable carbon isotopic signatures. Box plots show the maximum value, minimum value, median value, interquartile range, and outliers for benzenehexacarboxylic acid (B6CA), benzenepentacarboxylic acid (B5CA), and dissolved organic carbon (SPE-DOC). The stable carbon isotopic (δ 13 C) values are relative to Vienna Pee Dee Belemnite (VPDB). Source data are provided as a Source Data file Full size image At both the Atlantic and Pacific Ocean sites, DOC concentrations were highest in surface waters (63 and 81 μM-C, respectively), reached minima at depth (≥1000 m; ~42 μM-C; Fig. 3a ), and were in line with profiles previously reported for these locations [18] . SPE-DOC δ 13 C values were similar among oceanic samples (average = −22.9 ± 0.4‰; Fig. 2 ; Table 1 ) and consistent with oceanic DOC being derived from a marine phytoplankton source [16] . The majority of DOC released from phytoplankton is termed labile as it is rapidly degraded before it can accumulate [37] . DOC that persists for weeks to years is termed semilabile and is observationally defined as the pool of DOC which accumulates in surface waters, but does not survive over the longer timeframes required to mix into the deep ocean [18] . Semilabile DOC is enriched in hydrolysable sugars and other products of recent biological production [38] , but depleted in aromatic components [13] . It is this semilabile DOC which contributes to the DBC-depleted, DOC-enriched surface waters observed here (Fig. 3a, c ). In the deep ocean (>1000 m depth), DOC concentrations are low [18] (Fig. 3a ) and 14 C-depleted relative to DOC in surface waters [16] . Thus, DOC in the deep ocean is termed refractory as it appears to persist for thousands of years, becoming mixed throughout the global ocean [18] . In contrast to bulk DOC, DBC concentrations did not vary with depth (Fig. 3b ), consistent with the apparent refractory nature and long-term stability of DBC in the ocean [14] . The refractory DOC pool is one of the largest organic carbon stores on Earth and the largest in the ocean [18] , thus investigating its persistence is of major scientific interest and societal importance [37] . Since DBC appears to be representative of this refractory DOC [13] , a critical step in this endeavor is to constrain sources of oceanic DBC. Fig. 3 Atlantic and Pacific Ocean depth trends. Depth versus a dissolved organic carbon (DOC) concentration, b dissolved black carbon (DBC) concentration, c DBC:DOC ratio, and d ratio of benzenehexacarboxylic acid to pentacarboxylic acid (B6CA:B5CA) are shown for samples collected at Atlantic Ocean (light grey diamonds) and Pacific Ocean (dark grey triangles) sites. Source data are provided as a Source Data file Full size image In contrast to bulk DOC, DBC concentrations did not vary with depth (Fig. 3b ), but were higher, on average, in the Atlantic (0.76 ± 0.03 μM-C) than in the Pacific Ocean (0.61 ± 0.02 μM-C; p = 0.0001; Table 1 ). The Atlantic Ocean constitutes 24% of the global ocean volume but receives half of global freshwater discharge, while the Pacific Ocean constitutes 51% of the total ocean and receives only 20% of global freshwater discharge [39] . Lignin, an unambiguous molecular tracer for higher plant-derived material and terrestrial DOC, is also higher in the Atlantic Ocean compared to the Pacific Ocean [40] , [41] , [42] . Higher concentrations of lignin in the Atlantic Ocean have been ascribed to the greater relative proportion of river water received by this ocean basin [40] , [41] , [42] . Concentrations of DBC in rivers were roughly two orders of magnitude higher than in the ocean (Table 1 ). Consistent with previous studies [11] , [14] , [43] , DBC in rivers constituted a greater proportion of bulk DOC (6–9%) and exhibited a more condensed aromatic signature (higher B6CA:B5CA) than in the ocean samples, where DBC comprised <2% of DOC and had lower B6CA:B5CA values (Table 1 ). BPCA-specific δ 13 C values revealed a stark contrast in the isotopic composition of DBC in global rivers and the ocean (Fig. 2 ). Mean δ 13 C values for ocean B6CA and B5CA were −24.28 ± 1.62‰ and −22.88 ± 2.19‰, respectively. Taken together, mean BPCA-specific δ 13 C values were statistically similar between Atlantic and Pacific Ocean sites (B6CA, p = 0.20; B5CA, p = 0.48; Table 1 ). On average, BPCAs derived from oceanic DBC were significantly more enriched in 13 C (by ~6‰) than BPCAs derived from riverine DBC ( p < 0.0001; Fig. 2 ). In rivers, B5CA- and B6CA-specific δ 13 C values were significantly correlated ( R 2 = 0.74, p = 0.0003) and B5CA was consistently more enriched in 13 C than B6CA (Fig. 4 ). The isotopic offset between B5CA and B6CA in rivers ranged from 0.82 to 2.35‰ (Table 1 ). In contrast, δ 13 C values for oceanic B5CA and B6CA were not linearly related ( R 2 = 0.43, p > 0.05; Fig. 4 ), and the isotopic offset between B5CA and B6CA ranged from −2.11 to 4.95‰ (Table 1 ). The correlation between B5CA and B6CA δ 13 C values in rivers was expected, since we presume both molecular markers to be derived from the same pool of fire-derived condensed aromatics originating from soil BC. The observed difference between B5CA and B6CA δ 13 C values could be an intrinsic property of riverine DBC, thus providing further support for non-riverine sources of oceanic DBC. However, further research is required to elucidate specific biogeochemical mechanisms which control BPCA δ 13 C offset values in terrestrial and marine environments. Based upon our current results, hydrology and watershed land cover accounted for ~2‰ variability in riverine endmember DBC δ 13 C values (Table 1 ; Fig. 2 ). Oceanic BPCA-specific δ 13 C signatures were generally conserved with depth (Table 1 ), however B6CA was significantly depleted in 13 C (~2‰ lower) at 110 m depth in the Pacific Ocean ( p < 0.01) and B5CA was significantly depleted in 13 C (~2‰ lower) at 2000 m depth in the Atlantic Ocean ( p < 0.05). Overall, BPCA-specific δ 13 C values for different ocean water masses varied by only ~2‰ (Table 1 ; Fig. 2 ). Thus, endmember variability alone cannot account for the large isotopic discrepancy observed between BPCAs in rivers and the ocean. As such, our results indicate a non-riverine source for DBC quantified in the open ocean. Fig. 4 Relationship between compound-specific isotopic values. The stable carbon isotopic composition (δ 13 C) of benzenepentacarboxylic acid (B5CA) was plotted against that of benzenehexacarboxylic acid (B6CA) for samples collected from rivers (green circles) and the ocean (blue diamonds). Linear regressions are denoted by dotted lines and were B5CA δ 13 C = 1.09 × B6CA δ 13 C + 4.21 ( R 2 = 0.74; p = 0.0003) for riverine samples and B5CA δ 13 C = −0.46 × B6CA δ 13 C − 34.05 ( R 2 = 0.43; p > 0.05) for oceanic samples. Error bars represent propagated error associated with isotopic calibration or replicate error (1 SD), whichever is larger. The δ 13 C values are relative to Vienna Pee Dee Belemnite (VPDB). Source data are provided as a Source Data file Full size image Riverine and oceanic DBC isotopic discrepancy implications The application of BPCA-specific δ 13 C analysis for constraining sources of oceanic DBC assumes riverine BPCA-specific δ 13 C values are not fractionated (altered) as DBC transits coastal waters. Photochemical degradation has been shown to alter and remove DBC in natural waters [44] , [45] . Exposure to sunlight results in a photochemically processed DOC pool that is relatively enriched in 13 C [46] , [47] , due to the preferential loss of aromatic, 13 C-depleted DOC compound classes (e.g., lignin [48] ). However, BPCA-specific isotopic analyses bypass the molecular heterogeneity of bulk DOC to target individual compound classes (e.g., condensed aromatics [21] ). Therefore, exposure of DBC to sunlight is expected to degrade condensed aromatics similarly, where one carbon isotope is not preferentially photomineralized over another ( 12 C versus 13 C) within the same compound class. In the current study, lower DBC:DOC and B6CA:B5CA values observed for shallow ocean depths (Fig. 3c, d ) is consistent with photodegradation of DBC in sunlit surface waters [44] . BPCA-specific δ 13 C signatures in sun-bleached surface waters and the dark abyssal ocean were statistically identical (Table 1 ; p > 0.05), suggesting photochemistry has minimal-to-no impact upon DBC δ 13 C values. However, the impact of sun exposure upon riverine BPCA-specific δ 13 C signatures must be directly tested to confirm isotopic stability during photodegradation of DBC. If the physical removal of DBC from the water column (e.g., sorption to sinking particles [49] ), was primarily responsible for the observed offset between riverine and oceanic DBC δ 13 C values, then we would expect a gradient in δ 13 C values with depth in the ocean. However, the δ 13 C signature of oceanic DBC was fairly consistent with depth (Table 1 ). We look to Δ 14 C assessments for further insight on marine DBC cycling [14] , [43] . The apparent radiocarbon age of BPCAs increases in the deep ocean, suggesting the deep oceanic DBC pool is older (up to 23,000 14 C-years) and more refractory than the younger DBC (4,800 14 C-years) in the surface ocean [14] , mirroring trends observed for bulk DOC in the oceans [18] . The relative consistency of DBC δ 13 C signatures down-profile and similarity of BPCA-specific δ 13 C values between Atlantic and Pacific Ocean sites (Table 1 ) suggests a common source for modern DBC in the surface ocean and ancient DBC in the abyssal ocean. Assuming degradation processes do not result in a 13 C-enriched DBC pool, then isotopic trends for DBC match those for bulk DOC, where δ 13 C signatures indicate oceanic DOC to be dominated by marine sources with minimal contributions from terrestrial DOC [15] , [20] , [50] . Since our data are inconsistent with a riverine source for oceanic DBC (Fig. 2 ), we consider other sources of BPCAs to the open ocean. BPCA-specific δ 13 C values are similar to SPE-DOC δ 13 C values (Table 1 ), phytoplankton biomass, bulk marine DOC, and marine particulate organic carbon [16] . Based upon the isotopic signatures alone, a simple hypothesis is that the carbon in DBC, like bulk DOC, was originally fixed by phytoplanktonic production in the surface ocean. However, evidence for the autochthonous production of DBC in ocean waters does not exist and remains an area open for investigation. Biotic processes are proposed to alter the chemistry or diversity of freshly produced phytoplanktonic DOC, eventually resulting in the refractory pool of DOC observed in the ocean [51] . However, specific mechanisms which control the composition and reactivity of molecules which comprise the oceanic refractory DOC pool remain elusive [52] . Abiotic processes alter DOC, and likely also DBC, in the ocean. For instance, BPCAs could derive from organic material thermally processed or released by hydrothermal vents [53] . Hydrothermal vent conditions have also been shown to degrade refractory DOC in seawater [54] . Therefore, the net effect of these geothermally active hot spots on deep ocean DBC should be further investigated. The highly condensed (graphitic) BC contained in marine sediments is ancient (has a fossil Δ 14 C value), terrestrial in origin, and has a marine-like δ 13 C signature (−19 to −21‰), consistent with BC derived from bedrock erosion on land [55] . Petrogenic organic carbon constitutes ~20% of riverine particulate organic carbon exported globally [56] and has been shown to produce BPCAs upon oxidation [57] . Therefore, the dissolution of petrogenic BC from sinking particles or resuspended marine sediments could be another, yet unidentified, source of 14 C-depleted, 13 C-enriched BPCAs in the abyssal ocean. The derivation of BPCAs from petrogenic material suggests that B5CA and B6CA may not be exclusively representative of fire-derived organics [58] . The nitric acid reaction which converts organic matter to BPCAs is complex and lacks a systematic pattern for the oxidation of condensed aromatics [59] . Thus, nonpyrogenic sources of marine DBC may be possible, but remain unproven. Non-riverine, allochthonous sources of condensed organics which align with observed isotopic signatures may also contribute to the marine DBC pool. For instance, the atmospheric deposition of combustion-derived aerosols has recently been identified as the second-largest flux of DBC to marine surface waters (2 Tg-C per year) [60] . Globally, BC aerosols are derived roughly equally from both fossil fuel and biomass combustion processes [61] . However, contributions of fossil carbon to BC aerosols vary dramatically, ranging from ~10 to ~90% depending on geographic location and time of year [62] , [63] , [64] , [65] , [66] . While there is evidence that aerosol BC δ 13 C signatures are modulated by biomass type and combustion conditions, the isotopic composition of the charred precursor material is largely retained [67] . Global isotopic assessments of atmospheric BC do not exist, but δ 13 C values for BC aerosols over South Asia were shown to vary by up to ~4‰ and within the range observed for oceanic DBC [62] . In addition, BC in south Atlantic sediments exhibit a δ 13 C signature that is slightly enriched (−23 to −26‰) [68] compared to riverine DBC measured here (Fig. 2 ). Based upon these limited data, it is possible that aerosol-derived DBC has enriched δ 13 C signatures that could balance the observed discrepancy between riverine and marine DBC pools. However, a globally representative sample set is needed to constrain the isotopic signature of oceanic DBC sourced from pyrogenic aerosols. Rivers efficiently mobilize DBC from the land [11] , but mass balance estimates and our stable carbon isotopic signatures suggest most of this fire-derived material does not persist in the open ocean. Our findings are consistent with previous observations for the lack of bulk terrigenous dissolved organic matter in the ocean [19] . No information is available on the behavior of DBC as it transits estuarine and coastal zones, highlighting a critical area of research needed to fully understand connections between riverine and oceanic DBC pools. Further research is also needed to probe the stability of DBC δ 13 C signatures during photo-exposure and other processes, including sorption/desorption. Riverine export and atmospheric deposition deliver DBC to the ocean in excess of the apparent turnover of oceanic DBC [11] , [14] , [60] . Our isotopic data indicate additional, marine-derived sources are also likely. Thus, if BPCAs represent a biogeochemically coherent pool of compounds, then oceanic DBC turnover rates must be significantly faster than radiocarbon dating suggests [14] . Similarities between BPCA-specific and SPE-DOC δ 13 C values (Fig. 2 ) raise questions as to whether the BPCA method is capable of identifying sources of non-pyrogenic organic material. If δ 13 C fractionation during DBC removal processes is indeed negligible, then we will need to reexamine whether these condensed aromatic compounds truly represent the impact of fire upon the chemistry of the ocean, and search for new mechanisms which form this increasingly enigmatic molecular class. Sample collection Pacific Ocean samples were collected from Station ALOHA (22.45°N, 158.00°W) during the Hawaii Ocean Time-series (HOT) 301 cruise aboard the R/V Ka`imikai-O-Kanaloa . Samples from surface and mesopelagic depths (5, 110, 765, and 1000 m) were obtained from two casts on April 17, 2018 and the deep water sample (3500 m) was collected on April 18, 2018. Atlantic Ocean samples were collected from Hydrostation S (31.67°N, 64.17°W) during the Bermuda Atlantic Time Series (BATS) 358 cruise aboard the R/V Atlantic Explorer . Water samples were collected along a depth profile (1, 70, 2000, and 3000 m) on April 8, 2019. All seawater samples were collected using Niskin bottles mounted to the CTD rosette. For each sample, ~10 L was passed, by gravity, through a pre-cleaned in-line capsule filter (Whatman Polycap; 0.2 μm) into acid-cleaned Nalgene fluorinated HDPE carboys and pre-combusted glass vials and acidified to pH 2 using HCl prior to solid phase extraction and DOC analysis. River samples were collected from the main stem of the Amazon, Congo, Northern Dvina, Kolyma, and Mississippi Rivers, upstream of the river mouth where marine inputs were not observed (salinity = 0). The Amazon River is the largest river on Earth, drains the world’s largest tropical rainforest, and represents a major link in the transfer of carbon between land and sea [69] , [70] . One surface water sample was collected from the Amazon River near Óbidos (Brazil; April 20, 2018; 1.92°S, 55.53°W). The Congo River, located in equatorial Africa, is the second largest river on Earth [23] , [34] and was sampled from a site upstream of the cities of Kinshasa–Brazzaville on the main stem (DR Congo; 4.18°S, 15.21°E). Five samples were collected from the Congo River between August 2011 and April 2012, where discharge ranged from 23,740 to 54,120 m 3 s −1 , to account for potential hydrologically driven variations in DBC isotopic composition in a low latitude, subtropical river. The Northern Dvina River watershed is located in northwestern Russia, primarily drains low relief peatlands, is not underlain by permafrost [35] , and is a major contributor to pan-Arctic terrestrial DOC fluxes [24] . Four samples were collected from the Northern Dvina River in Arkhangelsk (64.55°N, 40.51°E) between October 2013 and May 2016, where discharge ranged from 637 to 13,380 m 3 s −1 , to capture isotopic variations in a high latitude river with extremely variable hydrology. The Kolyma River discharges into the Arctic Ocean and is a large, northern high-latitude river system that is, in contrast to the Northern Dvina, completely underlain by continuous permafrost [25] , [35] . One sample was collected from the Kolyma River, upstream of the city of Cherskiy (August 30, 2015; 68.75°N, 161.29°E). The Mississippi River drainage basin spans ~40% of the conterminous United States and contains one of the most productive agricultural regions in the world [26] , [33] . One sample was collected from the Belle Chase Ferry Landing on the Mississippi River, just south of New Orleans, LA (USA; February 23, 2016; 29.82°N, 90.00°W). All river samples were collected in situ using an oil-free pump equipped with a pre-cleaned, in-line capsule filter (Whatman Polycap, 0.2 μm) directly into acid-cleaned Nalgene bottles and pre-combusted glass vials. Samples were acidified to pH 2 using HCl prior to solid phase extraction and DOC analysis. DOC analysis and solid phase extraction Filtered and acidified samples were analyzed for DOC, measured as nonpurgable organic carbon using a Shimadzu TOC-L CPH analyzer equipped with an ASI-L autosampler. Sample DOC was quantified using a calibration curve made with a potassium hydrogen phthalate stock solution. Measurement accuracy and reproducibility was assessed by analyzing deep seawater and low carbon water reference materials obtained from the Consensus Reference Material (CRM) project (https://hansell-lab.rsmas.miami.edu/consensus-reference-material/index.html). Analyses of CRM were within 5% of reported values. DOC was isolated from samples via solid phase extraction (SPE; Varian Bond Elut PPL cartridges, 1 g, 6 mL) [27] prior to DBC analysis. Briefly, SPE cartridges were conditioned with methanol, ultrapure water, and acidified water. Filtered and acidified samples were passed through the SPE cartridges by gravity. Isolated DOC was then eluted from the SPE cartridges with methanol and stored at −20 °C until DBC analysis. Recovery of DOC by SPE was 74% for riverine and 48% for oceanic samples, on average (all data are provided in the Supplementary Dataset ). DOC recoveries in the current study are consistent with those observed previously for fresh and marine waters [27] . DBC quantification Sample DBC was quantified using the BPCA method, which chemically degrades condensed aromatic compounds into benzenehexacarboxylic acid (B6CA) and benzenepentacarboxylic acid (B5CA) molecular markers [28] . BPCAs were oxidized and quantified following previously described methods [21] , [28] . Briefly, aliquots of SPE-DOC (~0.5 mg-C equivalents) were transferred to 2 mL glass ampules and dried under a stream of argon until complete evaporation of methanol. Concentrated HNO 3 (0.5 mL) was added to each ampule, then ampules were flame-sealed and heated to 160 °C for 6 h. After oxidation, ampules were opened and HNO 3 was dried at 60 °C under a stream of argon. The BPCA-containing residue was re-dissolved in dilute H 3 PO 4 for subsequent analysis by high performance liquid chromatography (HPLC). Quantification of BPCAs was performed using a Dionex Ultimate 3000 HPLC system equipped with an autosampler, pump, and diode array detector. B6CA and B5CA were separated on an Agilent Poroshell 120 phenyl-hexyl column (4.6 × 150 mm, 2.7 µm) using an aqueous gradient of H 3 PO 4 (0.6 M; pH 1) and sodium phosphate (20 mM; pH 6) buffers [21] . BPCAs were quantified using calibration curves for commercially available B6CA and B5CA using a 5 mM BPCA-C stock solution. River samples were oxidized and analyzed in duplicate. Ocean samples were oxidized and analyzed in triplicate. The average coefficients of variation for replicate measurements of B6CA and B5CA were <5%. Sample DBC concentrations were calculated using the established power relationship between DBC (µM-C) and the sum of B6CA and B5CA (nM-BPCA) shown below ( n = 352, R = 998, p < 0.0001): [DBC] = 0.0891 × ([B6CA + B5CA]) 0.9175 [71] . DBC concentrations calculated using this equation are directly comparable to those measured in previous studies [10] , [11] . Stable carbon isotopic analyses Riverine and oceanic SPE-DOC methanol extracts were transferred to smooth-walled tin capsules (~0.25 mg-C per capsule) and methanol evaporated to dryness in an oven set to 60 °C. Sample-containing tin capsules were folded and combusted using a Thermo Scientific Flash EA Isolink CNSOH interfaced with a Thermo Scientific Delta V Plus IRMS. The δ 13 C composition of each sample was calibrated against an internal lab organic matter reference material (chitin from shrimp shells), which was previously calibrated against NIST glutamic acid (RM 8573) and sucrose (RM 8542) primary isotope reference standards. The 13 C content is expressed in δ 13 C per mil (‰) notation relative to Vienna Pee Dee Belemnite (VPDB). River samples were measured in duplicate and ocean samples were measured in triplicate. The standard deviation of replicate EA-IRMS measurements was <0.1‰. Compound-specific stable carbon isotopic values for individual BPCAs were measured using a Dionex Ultimate 3000 HPLC connected to a Delta V IRMS via an LC Isolink interface following methods detailed previously [21] . Online oxidation quantitatively converts baseline-separated BPCAs to CO 2 . 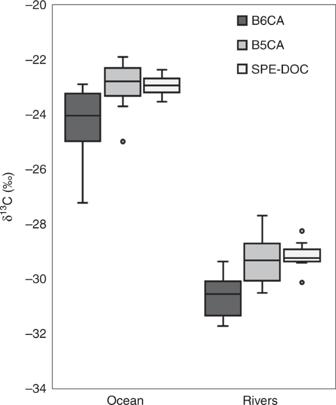Fig. 2 Riverine and oceanic stable carbon isotopic signatures. Box plots show the maximum value, minimum value, median value, interquartile range, and outliers for benzenehexacarboxylic acid (B6CA), benzenepentacarboxylic acid (B5CA), and dissolved organic carbon (SPE-DOC). The stable carbon isotopic (δ13C) values are relative to Vienna Pee Dee Belemnite (VPDB). Source data are provided as a Source Data file BPCA-derived CO 2 is then extracted from the mobile phase and dried prior to detection by IRMS. The δ 13 C values for B5CA and B6CA standards were measured by EA-IRMS following the same procedure described above to calculate and correct for offsets in HPLC-IRMS δ 13 C measurements [21] . River samples were analyzed in duplicate and ocean samples were analyzed in triplicate. Standard deviations applied to corrected sample δ 13 C values were propagated to account for errors associated with replicate EA-IRMS standard BPCA measurements, HPLC-IRMS standard BPCA measurements, and HPLC-IRMS sample BPCA measurements. The 13 C content is expressed in δ 13 C per mil (‰) notation relative to Vienna Pee Dee Belemnite (VPDB). 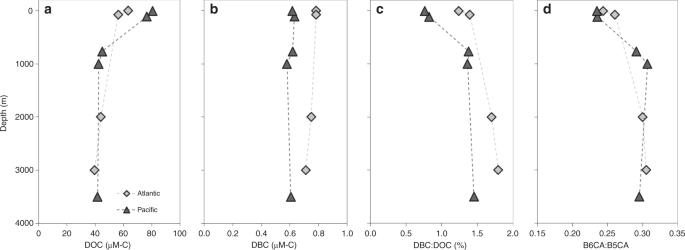Fig. 3 Atlantic and Pacific Ocean depth trends. Depth versusadissolved organic carbon (DOC) concentration,bdissolved black carbon (DBC) concentration,cDBC:DOC ratio, anddratio of benzenehexacarboxylic acid to pentacarboxylic acid (B6CA:B5CA) are shown for samples collected at Atlantic Ocean (light grey diamonds) and Pacific Ocean (dark grey triangles) sites. Source data are provided as a Source Data file 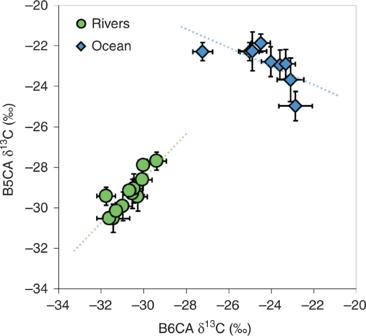Fig. 4 Relationship between compound-specific isotopic values. The stable carbon isotopic composition (δ13C) of benzenepentacarboxylic acid (B5CA) was plotted against that of benzenehexacarboxylic acid (B6CA) for samples collected from rivers (green circles) and the ocean (blue diamonds). Linear regressions are denoted by dotted lines and were B5CA δ13C = 1.09 × B6CA δ13C + 4.21 (R2= 0.74;p= 0.0003) for riverine samples and B5CA δ13C = −0.46 × B6CA δ13C − 34.05 (R2= 0.43;p> 0.05) for oceanic samples. Error bars represent propagated error associated with isotopic calibration or replicate error (1 SD), whichever is larger. The δ13C values are relative to Vienna Pee Dee Belemnite (VPDB). Source data are provided as a Source Data file The error associated with corrected δ 13 C values was typically <0.5‰. Statistical evaluations Significant variations in BPCA-specific and SPE-DOC δ 13 C values among rivers were determined using a one-way ANOVA. Tukey’s HSD tests were used to probe whether two isotopic values were significantly different (e.g., Congo versus Northern Dvina River SPE-DOC δ 13 C values, comparing δ 13 C values between oceanic water masses). An unpaired t test was used to compare mean riverine and oceanic BPCA-specific and SPE-DOC δ 13 C values. The above-described statistical evaluations assume normal distributions among data subsets. Linear regressions were used to assess the relationship between B6CA- and B5CA-specific δ 13 C values in riverine and oceanic datasets. Reporting summary Further information on research design is available in the Nature Research Reporting Summary linked to this article.